Direct printing of nanostructures by electrostatic autofocussing of ink nanodroplets Nanotechnology, with its broad impact on societally relevant applications, relies heavily on the availability of accessible nanofabrication methods. Even though a host of such techniques exists, the flexible, inexpensive, on-demand and scalable fabrication of functional nanostructures remains largely elusive. Here we present a method involving nanoscale electrohydrodynamic ink-jet printing that may significantly contribute in this direction. A combination of nanoscopic placement precision, soft-landing fluid dynamics, rapid solvent vapourization, and subsequent self-assembly of the ink colloidal content leads to the formation of scaffolds with base diameters equal to that of a single ejected nanodroplet. The virtually material-independent growth of nanostructures into the third dimension is then governed by an autofocussing phenomenon caused by local electrostatic field enhancement, resulting in large aspect ratio. We demonstrate the capabilities of our electrohydrodynamic printing technique with several examples, including the fabrication of plasmonic nanoantennas with features sizes down to 50 nm. A large pallet of techniques has been explored in the past few decades for nanofabrication, including powerful approaches such as photo- and electron-beam lithography, focussed-ion beam milling as well as nanoparticle-based self-assembly [1] , [2] , [3] , [4] , [5] , [6] , [7] . A particularly attractive approach is printing by ink jet [4] , electrohydrodynamics [1] , [5] , [7] , [8] and related techniques [2] , [3] , in which a nanoparticle-laden ink is dispensed from a scanning nozzle. Although these strategies provide flexible and inexpensive fabrication platforms, various physical and experimental processes have limited their resolution. Electrohydrodynamic (EHD) liquid ejection, well known from its use in electro-spinning [9] and -spraying [10] , has recently been employed in microfabrication for the production of defined planar entities of the order of a micrometre [1] , [7] . EHD ejection of liquid from a pipette nozzle is induced by the relaxation of ions to the liquid surface, on activation by an electric field. The ions are naturally present in the liquid (same amount of positive and negative species) and are its electrically conductive species. The induced electric stresses at the liquid–air interface can ultimately overcome the resisting effect of surface tension, causing liquid ejection. Depending on the direction of the electric field, either an excess of positive or negative ions will drive the ejection of liquid and attribute to its non-zero electric charge. Whereas different EHD ejection modes have been identified [11] , most related applications, including those related to microfabrication [1] , [7] , are based on the so-called cone-jet ejection mode in which a thin jet is released from the tip of a larger sharply converging liquid cone at high volume flow rates [10] , [11] , [12] . Another mode of ejection, called microdripping [5] , [11] , [12] , results in the periodic ejection of single, micron-sized spherical droplets from the apex of a larger steady liquid meniscus. Here we downscale this mode to the regime of nanodripping, while avoiding clogging of the dispenser tip by a sufficient reduction of the nanoparticle concentration. We will show that after droplet impact and solvent vapourization, nanoparticles are uniformly distributed in an area essentially equivalent to the diameter of a single droplet. In addition, we take advantage of an electrostatic nanodroplet autofocussing (ENA) effect to generate high aspect ratio out of plane nanostructures, built from the nanoparticles contained in the individual nanodroplets. Working together, the capabilities of this process allow the realization of nanostructures of different geometries and materials, which have homogeneous lateral size equal to that of a single nanodroplet. 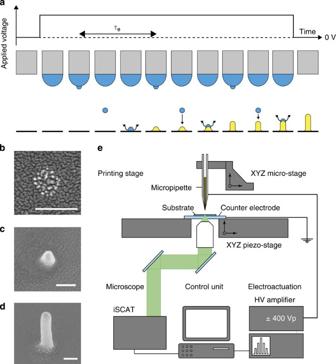Figure 1: Schematic of ENA printing process and set-up. (a) Growth of a liquid meniscus and subsequent ejection of ink nanodroplets from its apex on application of a DC voltage. During DC on-time, droplets are ejected at a homogeneous periodτeand, once impacted, are vapourized (represented by wavy arrows) in the course ofτe. After periodic repetition of this event (for illustration convenience merged into one cycle), a sharp structure consisting of a multitude of formerly dispersed nanoparticles rises from the substrate, attracting approaching charged droplets by ENA (straight arrows). The growth process is further illustrated with SEM micrographs (150 nm scale bar) of (b) the deposition pattern of a single nanodroplet and that of (c,d) actual nanopillars. (e) Schematic of the ENA NanoDrip set-up with the nozzle located above an underlying glass substrate placed on an ITO-coated glass slide representing the grounded counter electrode. Voltage stimuli were applied in the form of amplified DC signals between the ink-filled, metal-coated pipette and the counter electrode. A homebuilt iSCAT imaging system was used to detect printed structures. Working principle and set-up Figure 1a displays the essential steps in the temporal sequence of ENA NanoDrip printing. In the first step, a voltage is applied between the pipette/ink and a counter electrode, resulting in the generation of a meniscus and periodic ejection of ink nanodroplets from its lowest point. Once ejected, the nanodroplet is accelerated by the electric field towards the substrate where viscous effects pronounced by the nanodroplet size facilitate a soft landing and, owing to wetting-enhanced rapid vapourization, the droplet can dry during an ejection period τ e . Once the solvent has vapourized, the nanoparticles, formerly dispensed in the ink droplet, are found to be uniformly spread in an area corresponding to the projection of the spherical nanodroplet ( Fig. 1b ). Periodic occurrence of these events leads to a narrow accumulation of nanoparticles on the substrate. As this structure grows in height ( Fig. 1c,d ), its tip acts as a sharp electrode, creating strong electric-field gradients that focus the incoming droplets towards it and allow the structure to grow at a homogeneous diameter. The interval between voltage initiation and termination is denoted as pulse, as it has a defined duration and a sharp rise and fall ( Fig. 1a ). However, the pulse length does not influence the ejection frequency, nor the ejection process in general. The only purpose of using pulses is to precisely control the number of deposited droplets, that is, nanoparticles, and therewith the extent of printed nanostructures. It is worth stressing that our terminology of a pulse should not be confused with that of pulsed EHD jet-type processes reported by other authors [7] , [8] . In these studies, the pulse duration is related to the amount of liquid accumulated on the substrate, and is therefore an important process parameter affecting the lateral size of printed structures, after evaporation of the accumulated liquid. In contrast, the remarkable features of the nanodripping mode attained here, allow the solvent of each ejected and deposited droplet to be removed before the impact of the next one. The extent of accumulated liquid is therefore independent of the duration of the applied pulse. Figure 1: Schematic of ENA printing process and set-up. ( a ) Growth of a liquid meniscus and subsequent ejection of ink nanodroplets from its apex on application of a DC voltage. During DC on-time, droplets are ejected at a homogeneous period τ e and, once impacted, are vapourized (represented by wavy arrows) in the course of τ e . After periodic repetition of this event (for illustration convenience merged into one cycle), a sharp structure consisting of a multitude of formerly dispersed nanoparticles rises from the substrate, attracting approaching charged droplets by ENA (straight arrows). The growth process is further illustrated with SEM micrographs (150 nm scale bar) of ( b ) the deposition pattern of a single nanodroplet and that of ( c , d ) actual nanopillars. ( e ) Schematic of the ENA NanoDrip set-up with the nozzle located above an underlying glass substrate placed on an ITO-coated glass slide representing the grounded counter electrode. Voltage stimuli were applied in the form of amplified DC signals between the ink-filled, metal-coated pipette and the counter electrode. A homebuilt iSCAT imaging system was used to detect printed structures. Full size image The experimental set-up is shown schematically in Fig.1e and discussed in more detail in the Methods. The essential requirements and related physical mechanisms needed to achieve the nanodripping mode are also commented on in the Methods. If not specifically mentioned, the ink in all experiments consisted of a dispersion of 3–7 nm gold nanoparticles in n -tetradecane. The nozzle was fixed at a separation of 3–4 μm from the substrate, and a piezo-stage was used to position the substrate with nanometer accuracy at will. The printed structures were detected and imaged during deposition by an in-house-built microscope ( Fig. 1e and Methods). We remark, however, that the nanodroplets could not be detected during flight because of their large velocity magnitude of up to the order of 100 m s −1 ( Supplementary Methods and Supplementary Fig. S1 ). We used scanning electron microscopy (SEM) for a quantitative analysis of the nanoparticle patterns of a single droplet after deposition and solvent vapourization ( Fig. 1b ). For brevity, these patterns will be denoted as footprints in the following. Footprints are of crucial importance to ENA NanoDrip printing, because they allow the determination of the droplet size and ejection frequency. In addition, footprints help us understand the physical mechanisms behind the emergence of the resulting nanostructure geometries. Single footprints were obtained by fixing the nozzle in space while separating the sequential droplet impact positions through a sufficiently rapid movement of the substrate by the piezoelectric stage. With the knowledge of the substrate velocity and the spatial separation of footprints on the substrate, it is possible to evaluate an exact value for the ejection frequency ( Fig. 2a ). The lateral extent of footprints was found to approximately represent the droplet diameter. This unexpected result is based on an analysis of the volume of printed nanostructures ( Supplementary Fig. S2 ) in relation to the applied pulse length. Dividing the resulting ejection flow rate (ejected volume per pulse length) by the experimentally obtained ejection frequency yielded droplet sizes approximately matching the size of footprints ( Supplementary Fig. S3 and Supplementary Methods ). It is also found that the largest footprint diameters match the outer diameter of the employed pipette. As no other forces than the electric and surface tension forces are present (gravitation is negligible), the largest possible droplets are indeed expected to be similarly sized as the outer pipette diameter. Further reasoning that strengthens the equality argument of droplet and footprint sizes is provided later. 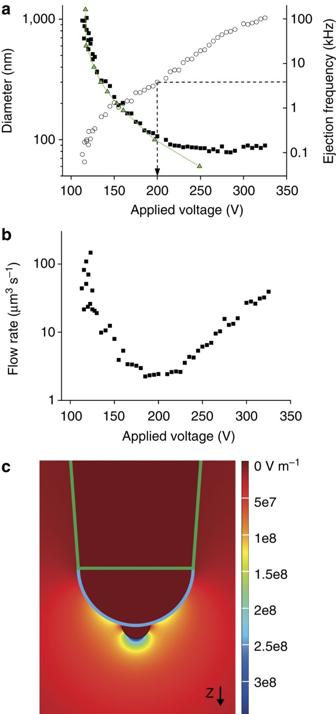Figure 2: Summary of measured and numerically derived key quantities for a 1.2 μm nozzle. (a) Experimentally obtained footprint diameter (full black squares) and ejection frequency (open circles) and numerically derived droplet diameter (full green triangles connected by straight green lines) as a function of applied voltage. The dashed arrow indicates the voltage threshold at which the charge relaxation time (τε) equals the ejection period (τe). Data points are based on up to 50 averaged values with standard errors below 5% (diameter) and 10% (frequency). The highest errors reach 10% (diameter) and 30% (frequency). (b) Flow rate of ejected fluid calculated from experimental footprint and frequency data. (c) Nozzle geometry used for numerical calculation of the electric force acting onto the liquid. The surface plot shows the calculatedz-component of the electric field around the modelled nozzle region during droplet ejection. The nozzle is depicted with a green line and the meniscus with a blue line. The image depicts a state in which the surface tension of the pendant droplet is matched by the electric stress and the droplet is therefore ready to be ejected. Figure 2: Summary of measured and numerically derived key quantities for a 1.2 μm nozzle. ( a ) Experimentally obtained footprint diameter (full black squares) and ejection frequency (open circles) and numerically derived droplet diameter (full green triangles connected by straight green lines) as a function of applied voltage. The dashed arrow indicates the voltage threshold at which the charge relaxation time ( τ ε ) equals the ejection period ( τ e ). Data points are based on up to 50 averaged values with standard errors below 5% (diameter) and 10% (frequency). The highest errors reach 10% (diameter) and 30% (frequency). ( b ) Flow rate of ejected fluid calculated from experimental footprint and frequency data. ( c ) Nozzle geometry used for numerical calculation of the electric force acting onto the liquid. The surface plot shows the calculated z -component of the electric field around the modelled nozzle region during droplet ejection. The nozzle is depicted with a green line and the meniscus with a blue line. The image depicts a state in which the surface tension of the pendant droplet is matched by the electric stress and the droplet is therefore ready to be ejected. Full size image Taking into account that footprints approximately represent the size of an ejected spherical droplet, their spatial extent could be employed to determine the size of droplets as a function of applied voltage ( Fig. 2a ). Combining frequency and size, the ejection flow rate could be determined ( Fig. 2b ). We find that with a nozzle of outer diameter ~1,200 nm, footprints as small as 80 nm were produced at an ejection frequency of several tens of kilohertz. To illustrate the homogeneous nature of frequency and droplet size in the nanodripping mode, we show in Supplementary Fig. S4 a series of separated footprints. These footprints are practically equidistant and of equal size. These and all other experiments were performed without active feedback control of the nozzle–substrate distance. That active feedback control is not a necessary requirement for a reproducible printing process is also confirmed by additional considerations and experiments on the sensitivity of the results on the distance between nozzle and substrate ( Supplementary Fig. S5 and Supplementary Methods ). Numerical and experimental analysis of the ejection process To estimate the diameter of the ejected droplets theoretically, we use a semi-numerical approach where we employ a simple geometrical model in which the small droplet to be ejected is pendant at the lower end of a hemispherical meniscus ( Fig. 2c ). On the basis of this model, we then calculate the forces acting onto the small droplet. Although the hemispherical meniscus shape has been observed before [5] , [12] , [13] , we experimentally verified that it develops with a similar shape also for the small nozzle sizes employed in our study ( Supplementary Fig. S6 ). Along this line, the size of the droplets can be predicted by a balance of electric and surface tension forces, whereby the electric force is calculated by the finite element method ( Fig. 2c shows the resulting electric field distribution) with the assumption that nozzle, meniscus and pendant droplet are all equipotential (see Methods ). Green symbols in Fig. 2a show the calculated droplet diameters as a function of the applied voltages. The agreement with the experimental data is very good up to the regime marked by the dashed arrow, where the liquid charge relaxation time τ ε (ratio of liquid permittivity and electrical conductivity) equals the ejection period, τ e , rendering the equipotential assumption invalid. We find that this regime change also corresponds to a minimum in the flow rate. For larger applied voltages, intensified electric stresses are produced at the meniscus, whereas charges cannot relax to the pendant droplet surface fast enough. As a result, a large liquid flow cannot be counteracted by a further reduction of the pendant droplet diameter, and the flow rate strongly increases for τ e below ~ τ ε . That we can reproduce both the evolution of the droplet diameter for τ e > τ ε and the divergence of experimental and theoretical data for τ e < τ ε is proof for the appropriateness of our simple semi-numerical model (within its limited applicability). It must be mentioned that the purpose of the theoretical estimate is not to reproduce the ejection dynamics (flow rate estimates are not possible). This task is highly complex and deserves a separate dedicated study, beyond the purpose of the present experimental work. Here we are only interested in a simple prediction of the size of ejected droplets, as direct observation was not possible. In Fig. 3a , we show, in addition to the footprint sizes of Fig. 2a , a second dataset where a nozzle with a diameter of 600 nm (half of that used before) was employed. It is found that the minimal ejection voltage (the voltage needed for ejecting a droplet with a diameter equal to that of the meniscus) decreases with decreasing nozzle diameter. In the Supplementary Methods , we illustrate theoretically the generality of this behaviour. Also plotted in Fig. 3a are numerical estimates of the droplet size. Evidently, the footprint diameters agree well with the theoretical estimates of the droplet size, confirming reproducibility of the numerical results. The presented data were then nondimensionalized by dividing the actual footprint diameter by the diameter of the meniscus, and by dividing the applied voltage by the minimal ejection voltage (see Supplementary Methods for reasoning). 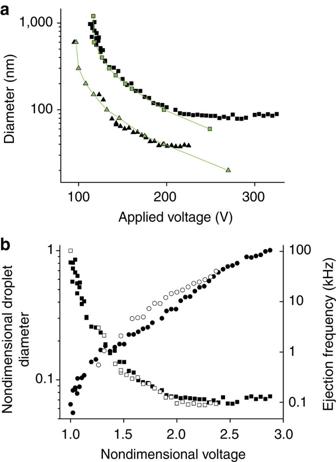Figure 3: Reproducibility with respect to different nozzle diameters. (a) Experimental (black symbols) and numerically (green symbols) derived footprint/droplet diameter for a 1.2-μm nozzle (squares, reprinted fromFig. 2) and a 600-nm nozzle (triangles). The minimal ejection voltage for the smaller nozzle was found to be ~20 V lower than that of the larger one. (b) The same experimental footprint data (squares) after nondimensionalizing (droplet size divided by nozzle size, applied voltage divided by minimal ejection voltage), with full symbols representing the large and open symbols representing the small nozzle. The fact that the datasets merge suggests that footprint sizes do indeed represent the droplet size, which is elucidated by additional experiments in theSupplementary Methods. We also plot the ejection frequency in absolute values (circles). At the same nondimensional voltage, frequencies observed for both nozzles, are about the same. This suggests an almost constant ejection frequency independent of the nozzle diameter. Figure 3b shows that the diameters of the nondimensional footprints are practically identical. In both cases, the smallest droplet size is ~1/15 of the nozzle size. The merging of the dimensionless datasets as well as the agreement of our numerical estimate with the experimental results substantially underpins the claimed equality of footprint and droplet diameter. In Fig. 3a , we also plot the dimensional ejection frequency as a function of nondimensional voltage. The ejection frequency seems to be nearly unaffected by the nozzle size variation, which implies that the flow rate at the same nondimensional voltage approximately scales with the droplet volume. At least for a droplet of the size of the meniscus, this may be understood by scaling the flow rate with the help of the classical Poiseuille equation ( Supplementary Methods ). Figure 3: Reproducibility with respect to different nozzle diameters. ( a ) Experimental (black symbols) and numerically (green symbols) derived footprint/droplet diameter for a 1.2-μm nozzle (squares, reprinted from Fig. 2 ) and a 600-nm nozzle (triangles). The minimal ejection voltage for the smaller nozzle was found to be ~20 V lower than that of the larger one. ( b ) The same experimental footprint data (squares) after nondimensionalizing (droplet size divided by nozzle size, applied voltage divided by minimal ejection voltage), with full symbols representing the large and open symbols representing the small nozzle. The fact that the datasets merge suggests that footprint sizes do indeed represent the droplet size, which is elucidated by additional experiments in the Supplementary Methods . We also plot the ejection frequency in absolute values (circles). At the same nondimensional voltage, frequencies observed for both nozzles, are about the same. This suggests an almost constant ejection frequency independent of the nozzle diameter. Full size image Nanostructure growth initiation The cyclic release and deposition of spherical droplets, one at a time, in nanodripping allows enough time for the efficient removal of solvent by vapourization during τ e . This lets nanoparticles of a multitude of footprints accumulate into a tight scaffold, which only increases in height while maintaining constant lateral size. This mechanism is in great contrast to that of cone-jet printing in which the ink and the accompanying nanoparticles continuously spread on the substrate owing to the high immediate volume flow rates [7] , [8] . Fast vapourization of a droplet implies that to avoid clogging at the nozzle, the volumetric rate of vapourization at a single deposited droplet must be higher than that at the meniscus itself ( Supplementary Methods ). Our experiments show that this is fulfilled, if the ink is able to sufficiently wet the substrate surface [14] . Indeed, the employed glass slips exhibited excellent wetting properties with contact angles <10°. In addition, we registered very strong wetting also when depositing optically observable volumes of solvent onto dried nanoparticle layers. This behaviour is expected due to the solvent-specific coating of the nanoparticles. In contrast to the outcome on wetting substrates (that is, nanopillars with homogeneous diameter), the deposition of droplets onto only partially wetted substrates (contact angle ~60°; see Methods ) resulted in nanoparticle scaffolds with spherical cap geometry several times larger than a single droplet ( Supplementary Fig. S7 ). Such a shape is clear evidence of a single drying sessile ink droplet containing mobile nanoparticles [15] and illustrates the accumulation of several smaller droplets on the substrate due to insufficient vapourization rates. An interesting and important feature of ENA NanoDrip printing is the lack of a coffee-stain effect [16] and the equality of droplet and footprint size despite strong wetting of the ink. The lack of a coffee-stain pattern can be explained by the low Peclet number in the range of unity [17] , giving rise to diffusion-dominated nanoparticle motion ( Supplementary Methods ). However, the small size of footprints requires further studies that go beyond our current work. We believe that the underlying mechanism of this unexpected behaviour is that size-related strong viscous damping causes a soft-landing process despite the high impact velocities ( Supplementary Fig. S8 and Supplementary Methods ) whereas electric forces are not found to notably enhance impact spreading ( Supplementary Table S1 and Supplementary Methods ). Hence, a droplet will initially be deposited on the substrate with a diameter similar to that of its spherical state, and only afterwards, capillarity-driven wetting will slowly increase its diameter [18] ( Supplementary Methods ). The observed equality of droplet and footprint sizes implies that, in our case, nanoparticle settling occurs before the longer wetting phase. However, since the time that a nanoparticle needs to diffuse along the droplet domain is similar to the expected wetting time, diffusion alone is not expected to allow full nanoparticle settling during the required timescale ( Supplementary Table S2 and Supplementary Methods ). We speculate that because of the small size of the deposited droplets, long-range particle-substrate forces, especially Coulomb forces, extend over the entire droplet domain, thus confining the particle settlement process [17] , [19] . The simultaneous presence of ionic charge and external electric field renders rigorous quantification difficult and requires further study. We note in passing that footprint patterns did not differ for nanodroplets of opposite charge. Structure growth by electrostatic nanodroplet autofocussing Once the first few droplets have laid the foundation of a pillar ( Fig. 1a ), the electrostatic field induced at its strongly curved surface focusses the following incoming nanodroplets to the tip of the forming pillar. Because of the zero lateral electric field component at the nozzle-substrate axis, droplets stay in a narrow path even when working at nozzle-substrate distances as high as ~5 μm (further increase in this separation can eventually lead to unfocussed structure growth; see Supplementary Fig. S9 ). 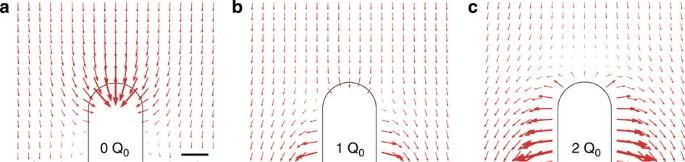Figure 4: Electrostatic field-focussing effect for charged and uncharged nanopillars. The images show nanopillars subjected to an applied electric field. The arrows point to the direction of acceleration of a charged nanodroplet with an arbitrary intensity represented by the arrow length. The figure compares the resulting field for three structures, bearing a residual charge of (a) 0, (b) 1 or (c) 2 droplets (Q0=unit droplet charge). Because residual charge acts repulsively to new approaching droplets, the field-focussing effect is overtaken by repulsion already for one residual droplet charge. This illustrates that also from the charging point of view, complete vapourization between consecutive droplet ejections is a requirement for ENA NanoDrip printing. Scale bar, 50 nm. Figure 4a–c show the results of electrostatic simulations for three scenarios of different residual ionic charge originating from the deposited charged droplets. The figures suggest that electrostatic autofocussing only acts on droplets in close proximity to a growing nanostructure and only if the deposited charge is sufficiently removed. Figure 4a represents the most optimal situation of full charge removal during the course of solvent vapourization. In this case, the metal structure clearly acts attractive on approaching nanodroplets. Simulation results for residual charge, equal to that carried by 1 droplet and 2 droplets, respectively, ( Fig. 4b,c , respectively) imply that, on a non-conductive substrate liquid- and concomitant-charge accumulation would lead to detrimental repulsion effects between pillar structure and approaching charged droplet. Thus, observation of high aspect ratio pillars, as that shown in Fig. 5a with 50-nm width and 850-nm height, confirms the need for rapid liquid vapourization carrying away ionic charge. In combination with the processes enabling uniform footprint patterns at the same size as a droplet, ENA leads to an equality of droplet and pillar diameter. We verified this important feature by analysing the diameters of nanopillars printed at a set of voltages and plotting them together with measured footprint sizes ( Supplementary Fig. S10 ). Figure 4: Electrostatic field-focussing effect for charged and uncharged nanopillars. The images show nanopillars subjected to an applied electric field. The arrows point to the direction of acceleration of a charged nanodroplet with an arbitrary intensity represented by the arrow length. The figure compares the resulting field for three structures, bearing a residual charge of ( a ) 0, ( b ) 1 or ( c ) 2 droplets ( Q 0 =unit droplet charge). Because residual charge acts repulsively to new approaching droplets, the field-focussing effect is overtaken by repulsion already for one residual droplet charge. This illustrates that also from the charging point of view, complete vapourization between consecutive droplet ejections is a requirement for ENA NanoDrip printing. Scale bar, 50 nm. 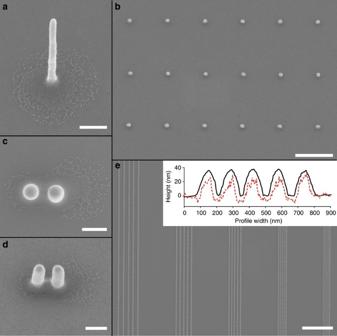Figure 5: SEM micrographs of printed nanostructures with dimensionalities from 0D to 2D. (a) Gold nanopillar of diameter ~50 nm and aspect ratio of ~17 (Scale bar, 200 mm). (b) Top and (c) side view of nanopillars printed subsequently at 200 nm center-to-center distance (scale bar, 200 nm). (d) 80-nm wide dots printed into a 1-μm lattice constant array (1 μm scale bar). (e) Printed tracks with pitch sizes of 250, 200, 150, 100 and 75 nm (scale bar, 2 μm). The inset shows AFM (full black lines) and SEM (red dashed lines) profiles of 150-nm pitch size. The height of AFM profiles is given in nanometers. The SEM profiles are in arbitrary units. Tracks have reproducible heights of ~40 nm and are well separated. Full size image Figure 5: SEM micrographs of printed nanostructures with dimensionalities from 0D to 2D. ( a ) Gold nanopillar of diameter ~50 nm and aspect ratio of ~17 (Scale bar, 200 mm). ( b ) Top and ( c ) side view of nanopillars printed subsequently at 200 nm center-to-center distance (scale bar, 200 nm). ( d ) 80-nm wide dots printed into a 1-μm lattice constant array (1 μm scale bar). ( e ) Printed tracks with pitch sizes of 250, 200, 150, 100 and 75 nm (scale bar, 2 μm). The inset shows AFM (full black lines) and SEM (red dashed lines) profiles of 150-nm pitch size. The height of AFM profiles is given in nanometers. The SEM profiles are in arbitrary units. Tracks have reproducible heights of ~40 nm and are well separated. Full size image The combination of small droplet trajectory divergence and electrostatic autofocussing allows not only a remarkable aspect ratio in the formation of nanostructures, but also a superb spatial control of structural placement as illustrated by an array of printed ~80-nm wide nanodots of 1 μm lattice constant ( Fig. 5b ). The deviation between the actual and aspired positions is in the range of only a few nanometers. The spacing between structures can be further reduced as shown by a pair of sequentially printed nanopillars of diameter 120 nm, separated by a gap of 80 nm ( Fig. 5c,d ). This example emphasizes that moving the central impact region by an amount as small as the structure diameter is sufficient to prevent droplets from being attracted to the previously printed nanopillar. The attainable positioning accuracy and resolution are further demonstrated in Fig. 5e with an example of printed in-plane tracks. These were created by introducing a constant relative movement between the nozzle and the substrate during droplet ejection. Figure 5e displays tracks at pitch sizes ranging from 75 nm to 250 nm, where full separation is achieved for track distances down to 100 nm. Atomic force microscopy profiles further reveal reproducible track heights of about 40 nm ( Fig. 5e , inset). Such tracks may be employed as electrical conductors. Supplementary Figure S11 provides an example of a printed track after an annealing treatment, proving that those structures do not loose integrity when being sintered but instead form one entity. Quantitative results on the electrical behaviour of printed tracks in relation to different annealing treatments will be dedicated to future studies. Flexibility towards growth direction and material Interestingly, ENA also allows fabrication of nanopillars at a variety of tilting angles, paving the way towards the formation of a wide palette of out-of-plane nanostructures. These tilted structures are created by a slow lateral movement of the piezo-stage during the deposition process. The resulting shift of the projected droplet impact position with respect to the apex of a growing nanostructure will induce ENA to bend the trajectory of the approaching droplet towards the nanostructure extremity. The direction at which a droplet impacts at the structure apex depends on the velocity of the stage movement and ultimately on the velocity at which the structure grows. For example, if the piezo-stage moves at half the structure growth velocity, the nanostructure will grow at a 45° tilting angle. This could be reproduced by growing tilted nanopillars at varying piezo-stage velocities, where the tilting angle was found to be proportional to the velocity of the substrate movement ( Fig. 6 ). 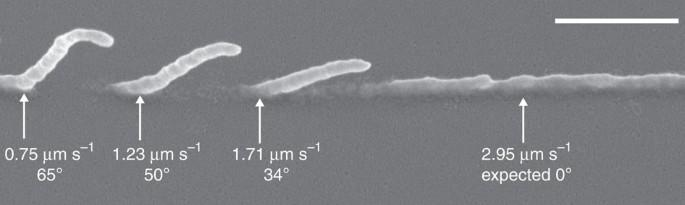Figure 6: Structures printed at varying substrate movement velocity. Tilted nanopillars generated by ejecting nanodroplets during relative nozzle-substrate movement at linearly increasing substrate velocities. Pillars have a diameter of ~55 nm (scale bar is 500 nm). The velocities and immediate pillar-tilting angles at the positions marked with an arrow are displayed in the SEM micrograph. It is found that the tilting angle is directly proportional to the employed substrate velocity. From this linear relationship, the structure growth velocity can be deduced, which is ~3 μm s−1. If the substrate movement is above 3 μm s−1, the pillars will merge with the substrate and generate a track. That the pillar already merges with the substrate at lower velocity is due to the non-zero pillar diameter and the still increasing velocity, which prohibit the pillar to elevate above the substrate. The separation between pillars is not induced manually, by briefly interrupting ejection, but occurs spontaneously during the process. This phenomenon may be related to the inhomogeneous nature of the electric vector field (Supplementary Discussion). Figure 6: Structures printed at varying substrate movement velocity. Tilted nanopillars generated by ejecting nanodroplets during relative nozzle-substrate movement at linearly increasing substrate velocities. Pillars have a diameter of ~55 nm (scale bar is 500 nm). The velocities and immediate pillar-tilting angles at the positions marked with an arrow are displayed in the SEM micrograph. It is found that the tilting angle is directly proportional to the employed substrate velocity. From this linear relationship, the structure growth velocity can be deduced, which is ~3 μm s −1 . If the substrate movement is above 3 μm s −1 , the pillars will merge with the substrate and generate a track. That the pillar already merges with the substrate at lower velocity is due to the non-zero pillar diameter and the still increasing velocity, which prohibit the pillar to elevate above the substrate. The separation between pillars is not induced manually, by briefly interrupting ejection, but occurs spontaneously during the process. This phenomenon may be related to the inhomogeneous nature of the electric vector field ( Supplementary Discussion ). Full size image Finally, we point out that ENA NanoDrip printing can be easily adopted for growth from materials other than gold or even nonmetals as long as their dielectric constants are higher than that of the surrounding medium. To demonstrate this, we have successfully printed nanopillars made of silver and zinc oxide ( Supplementary Fig. S12 ). ENA NanoDrip printing for plasmonics ENA NanoDrip printing paves the way for easy and versatile creation of a large variety of complex nanostructures. An application of particular interest in the past half-a-decade concerns metamaterials [20] and optical nanoantennas [21] made of plasmonic nanostructures in various shapes such as split ring, split-rod, bow-tie and so on. Currently, these structures can only be fabricated using e-beam lithography (EBL) or focussed-ion-beam (FIB) milling, both of which are very expensive and thus not available to many researchers. ENA NanoDrip printing promises to deliver the same performance for optical antennas and metamaterials. As an example, we have printed a so-called Yagi-Uda antenna (optical analogue of the old TV antennas). 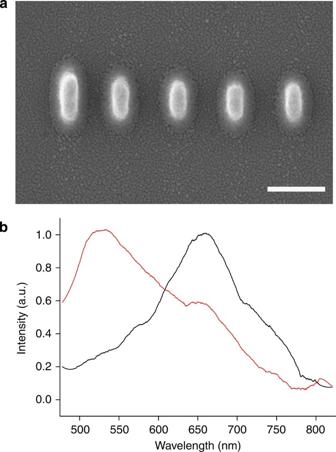Figure 7: ENA NanoDrip printing for plasmonic applications. (a) SEM micrograph of the ENA NanoDrip-printed geometry of a recently demonstrated Yagi Uda antenna22(scale bar, 200 nm). (b) The measured scattering spectrum of a printed and subsequently annealed gold nanopillar with a diameter of 50 nm and aspect ratio of ~4. The graph shows spectra for longitudinal (black line) and transverse (red line) excitation. The small peak at 660 nm for transverse polarization is due to slight coupling of the excitation into the longitudinal mode. Figure 7a displays a SEM image of this structure. An antenna using the same design parameters (structure size and separations) was recently realized using EBL and demonstrated a directional emission pattern [22] . Figure 7: ENA NanoDrip printing for plasmonic applications. ( a ) SEM micrograph of the ENA NanoDrip-printed geometry of a recently demonstrated Yagi Uda antenna [22] (scale bar, 200 nm). ( b ) The measured scattering spectrum of a printed and subsequently annealed gold nanopillar with a diameter of 50 nm and aspect ratio of ~4. The graph shows spectra for longitudinal (black line) and transverse (red line) excitation. The small peak at 660 nm for transverse polarization is due to slight coupling of the excitation into the longitudinal mode. Full size image Having mastered the required geometrical parameters, one might wonder whether the structures resulting from the assembly of small colloidal gold nanoparticle have proper plasmonic response. To investigate this, we have printed a nanopillar with a base diameter of 50 nm and height of 200 nm and annealed it at 260°C. In Fig. 7b , we plot the plasmon spectra recorded under illumination polarized perpendicular (transverse) and parallel (longitudinal) to the nanopillar long axis. Resonances at 528 nm and 660 nm are in reasonable agreement with the theoretical predictions of 525 nm and 700 nm, respectively [23] . The spectra before the annealing process deviate from these values and are found in the Supplementary Fig. S13 . We remark that recent works have shown that, in fact, structures as simple as single plasmonic nanospheres [24] , nanodisks [25] or nanorods [26] can act as optical antennas with strong scattering properties and large optical near-field enhancement [20] , [21] , [24] . Printing such plasmonic nanostructures may also be employed for applications in gas sensing [27] , graphene pholtovoltaics [28] or low-energy photon detection [29] . In this work, we have presented feature sizes down to 50 nm by using nozzle diameters in the range of 1 μm. Downscaling these by only a factor of 2–5 would make our method fully competitive with the state-of-the-art performances of EBL or FIB. Observed footprints, originating from a 600-nm nozzle, have already reached ~35 nm. Besides reducing the size of employed nozzles, even smaller droplets could be achieved by pinning the meniscus not at the outer, but at the inner opening [30] , for example, by treating the nozzle surface with a solvent-repelling coating [1] , [30] . This may allow droplets as small as 20 nm from a 600 nm nozzle at a manageable effort. Further downscaling may be achieved by employing ever smaller nozzles. Along this line, we believe that a lower limit to the process will mainly be induced by difficulties of further nozzle downscaling (also the involved clogging issues) or size restrictions imposed by the nanoparticles (as particles should still be substantially smaller than the structures they build). Of great importance for any technical advancement will also be a better understanding of the different physical aspects. We have identified several stringent conditions, which have to be fulfilled for proper functioning of ENA NanoDrip printing. Most important is a proper adjustment of the diverse flow rates, namely of ejection flow rate and vapourization flow rate at both, droplet and meniscus (see also the Supplementary Methods , concerning this topic). The implementation of strongly deviating solvents (for example, with respect to surface tension, viscosity, vapour pressure and so on) will not be successful at the same conditions used here. In this respect, it will be of importance to also include external factors that we have not yet investigated (for example, temperature). We believe that both downscaling and further process versatility will be accompanied with a better understanding of the process. In contrast to techniques like EBL and FIB, ENA NanoDrip printing is orders of magnitude less expensive, does not require vacuum, and can easily create out-of-plane structures. We anticipate that availability of reproducible microfabricated print heads [31] in the future will introduce further controllability and parallelization of the process with a multitude of nozzles, providing an on-demand, bottom-up and scalable nanofabrication technique. Printing process The set-up shown in Fig. 1a consists of an in-house built microscope equipped with a 3D piezo-stage (MadCityLabs), electrical equipment for pulse generation and a central control unit. A glass substrate was placed on top of an ITO coated glass slide mounted at the piezo-stage. The piezo-stage had a working distance of 300 μm. In the respective area, structures can be well aligned at the inherent precision of the piezo-stage (generally <10 nm). For optical detection, this microscope worked in the iSCAT mode [32] . This allowed highly sensitive detection of printed nanostructures and tight focussing (low view of depth). The latter was essential for controlling the nozzle-substrate distance (see below for more information). For the respective experiments, the wettability of the substrate with respect to the Au ink was reduced by vapour phase coating of a self-assembled monolayer of 1 H,1 H,2 H,2H-perfluorooctyltrichlorosilane, resulting in a contact angle of ~60°. Glass pipettes with outer diameters between 550 nm and 1,300 nm were prepared with a Sutter P-97 pipette puller. Only pipettes with good nozzle quality, that is, having no cracks, chipped edges or the like, were used. Ink was introduced to the backside opening of the pipette and drawn to the very tip by capillary forces without any applied pressure. The outer pipette wall and a small region of the nozzle tip interior were coated with a 10-nm adhesion layer of titanium followed by 100 nm of gold using e-beam evaporation. Irrespective of the small nozzle size, only minimal caution was necessary when handling them. The nozzle-substrate distance was assessed with a precision of about 150 nm by tightly focussing at the capillary tip and then moving the focal plane at a controlled distance by a movement of the micro-stage holding the objective. The substrate was then placed into focus by a z -movement of the piezo-stage. For most experiments, the employed ink contained 3–7 nm gold particles in cyclododecene (ULVAC Technologies). The ink was diluted by a factor of 50 with n -tetradecane to arrive at a final concentration of ~0.1 vol%. Dilution was necessary to avoid clogging, at least for a period of several minutes. At substantially higher concentrations, rapid clogging prohibited a smooth workflow. Early clogging could normally be reversed by the application of a high-voltage pulse (up to 400 V). For calculations, the physical properties of n -tetradecane were adopted. The measured conductivity of the diluted ink was 6.8×10 −8 Sm −1 . Silver (ULVAC Technologies) and zinc oxide (Nanograde) inks were both based on n -tetradecane and contained nanoparticles with sizes of 3–7 nm and ~25 nm, respectively. Voltage signals were generated by a waveform generator (RIGOL) and amplified by a homemade HV amplifier to up to 400 Volts. Annealing and optical measurements Thermal annealing was performed in a rapid thermal annealing oven (Jipelec). During purge-pumping by nitrogen gas, the temperature was first ramped at 2 °Cs −1 to 100 °C, then at 10 °Cs −1 to 200 °C and finally at 3 °Cs −1 to 260 °C. Once the temperature reached 260°C, the heat source was deactivated and a 5% mixture of H 2 /N 2 was introduced at 500 s.c.c.m. The sample was passively cooled to room temperature. Scattering spectra were obtained in a low grazing angle arrangement ( Supplementary Fig. S14 ). Requirements for the nanodripping mode To achieve the nanodripping mode, the characteristic time of supply of liquid to the droplet ( τ q ) has to be longer than the characteristic time of drop formation [11] . Here τ q is estimated as the duration between consecutive droplet ejections ( τ e ) and therefore equals the droplet volume (~ d 3 ) divided by the volume flow rate . The characteristic time of drop formation τ d is based on the intrinsic properties of the fluid with μ denoting the liquid viscosity and γ the liquid surface tension [11] The drop formation time states how long it takes for a liquid element, ejected through a circular exit with diameter d , to form a droplet solely by the action of surface tension and viscous resistance. If the characteristic time of supply of liquid is shorter than the drop formation time, the ensuing convective liquid flow will not allow for the relaxation of the liquid element into a droplet. Instead, a continuous jet can form, which would be the basis of the cone-jet ejection mode. A timeframe right before droplet ejection is schematically depicted in Fig. 2c , where the meniscus diameter is assumed to be equal to the outer nozzle diameter. During ejection, the meniscus has to be quasi-steady, which requires the charge relaxation time τ ε to be smaller than the time of supply of liquid to the meniscus τ Q (the latter is also given by equation (1) but with d replaced by the meniscus diameter D ). The charge relaxation time describes the process of relaxing charges on a conductor surface, that is, the time it takes for the surface potential to settle after a voltage stimulus and is defined as Here ε and σ are the liquid electric permittivity and conductivity. If the charge relaxation time is longer than the time of supply of liquid, more charge would be removed from the surface by liquid flow than what is delivered by bulk electrical conduction. The surface charge would therefore diminish causing the meniscus to inherently collapse. In Supplementary Fig. S15 a distribution of these important timescales is shown, proving that the requirements leading to nanodripping ejection are fulfilled for the entire regime investigated in this study. Numerical simulations Numerical simulations for the determination of the electric field were performed by COMSOL multiphysics software in the AC/DC electrostatics module, using the linear UMFPACK solver. The geometry of the pipette was determined from SEM micrographs and modelled as axisymmetric. The model of the nozzle region includes the pipette, a pulled liquid meniscus and a small pendant droplet at its tip, all of which are assumed to be at equipotential. The grid was automatically refined until results deviated by less than 2%. To estimate the droplet diameter, d , the following balance of surface tension and electric forces has to be fulfilled: Here γ represents the surface tension, E is the electric field, ε the permittivity of air and d a z a differential surface element for the integration over the small hemispherical surface with subscript z denoting the z -direction. A surface plot of the obtained electric field can be found in Fig. 2c . The integral in equation (4) was evaluated by solving for the Maxwell stress tensor in the z -direction followed by integration on the surface of the small pendant droplet. Input voltages were iteratively adjusted until the resulting electric force matched the surface tension force with an accuracy of better than 2%. How to cite this article: Galliker, P. et al . Direct printing of nanostructures by electrostatic autofocussing of ink nanodroplets. Nat. Commun. 3:890 doi: 10.1038/ncomms1891 (2012).